TRPA1 mediates spinal antinociception induced by acetaminophen and the cannabinoid Δ9-tetrahydrocannabiorcol TRPA1 is a unique sensor of noxious stimuli and, hence, a potential drug target for analgesics. Here we show that the antinociceptive effects of spinal and systemic administration of acetaminophen (paracetamol) are lost in Trpa1 −/− mice. The electrophilic metabolites N -acetyl- p -benzoquinoneimine and p -benzoquinone, but not acetaminophen itself, activate mouse and human TRPA1. These metabolites also activate native TRPA1 and, as a consequence, reduce voltage-gated calcium and sodium currents in primary sensory neurons. The N -acetyl- p -benzoquinoneimine metabolite L -cysteinyl- S -acetaminophen was detected in the mouse spinal cord after systemic acetaminophen administration. In the hot-plate test, intrathecal administration of N -acetyl- p -benzoquinoneimine, p -benzoquinone and the electrophilic TRPA1 activator cinnamaldehyde produced antinociception that was lost in Trpa1 −/− mice. Intrathecal injection of a non-electrophilic cannabinoid, Δ 9 -tetrahydrocannabiorcol, also produced TRPA1-dependent antinociception in this test. Our study provides a molecular mechanism for the antinociceptive effect of acetaminophen and discloses spinal TRPA1 activation as a potential pharmacological strategy to alleviate pain. The identification of TRPA1 as a sensor of noxious stimuli has contributed to the understanding of how chemical, thermal and mechanical stimuli trigger nociception in the periphery [1] , [2] , [3] , [4] , [5] . Chemical activation of TRPA1 produces pain, irritation and hyper-reactivity in skin and visceral organs [6] , [7] , [8] . Although there are indications that TRPA1 is present in the spinal cord [9] , its role in spinal processing of nociceptive input is not obvious. Acetaminophen (acetyl- p -aminophenol; APAP), also known as paracetamol, is a widely used analgesic and antipyretic agent, which in terms of adverse effects has well-recognized advantages over the non-selective cyclooxygenase (COX) inhibitors at therapeutic doses. Since the discovery of APAP more than a century ago, its mechanism of action has remained a mystery, although an action in the central nervous system, including the spinal cord, has been a recurrent claim [10] , [11] , [12] , [13] , [14] , [15] , [16] , [17] , [18] . The metabolism of APAP is complex and the effective dose is high and dependent on the species and route of administration [19] , [20] , [21] . Previous studies on APAP metabolites have largely focused on their toxic actions. However, our finding that APAP is metabolized by fatty acid amide hydrolase (FAAH) to N -(4-hydroxyphenyl)-5Z,8Z,11Z,14Z-eicosatetraenamide (AM404) and structurally related N -acylphenolamines in the rodent brain has drawn our attention to various metabolites of APAP as potential mediators of its therapeutic actions [22] , [23] . In initial studies, we found that the APAP metabolite p -aminophenol ( p -AP) could activate primary sensory neurons in vitro in a manner that did not depend on its conversion to N -acylphenolamines by FAAH. This effect as well as the breakdown of p -AP was prevented in the presence of the antioxidant ascorbic acid. These early experiments and the subsequent findings that TRPA1 is activated by electrophilic compounds [4] , [5] led us to speculate that p -AP and APAP indirectly activate TRPA1 on primary sensory neurons, after their conversion to electrophilic compounds such as p -benzoquinone ( p -BQ) and N-acetyl- p -benzoquinoneimine (NAPQI). The formation of these electrophilic compounds in vivo is catalysed by several enzymes, including cytochrome P450 (CYP450) monoxygenases, peroxidases and COX, many of which are present in the central nervous system [19] , [20] , [21] , [24] , [25] , [26] , [27] , [28] , [29] . NAPQI is believed to mediate the well-known hepato- and nephro-toxic effects of APAP. However, NAPQI metabolites, including L -cysteinyl- S -APAP, can be detected in human and mouse blood or urine after ingestion of therapeutic and non-toxic doses of APAP [19] , [24] , [26] . The finding of CYP450 monoxygenase and COX-2 activity and immunoreactivity in the rat and human spinal cord, including laminae I and II of the dorsal horn [28] , [29] , is of particular interest and raises the possibility that NAPQI is formed in regions of the spinal cord where the central terminals of TRPA1-expressing neurons are abundant. The ability of TRPV1 activators to produce spinal analgesia [30] , [31] and the coexpression of TRPV1 and TRPA1 on a subpopulation of nociceptive sensory neurons prompted us to examine whether the analgesic effect of APAP could involve the activation of TRPA1 located on the central terminals of primary afferent neurons. We, therefore, investigated the role of TRPA1 in the antinociceptive effect of intrathecal and systemic administration of APAP and determined whether electrophilic metabolites of APAP, such as NAPQI and p -BQ, produce antinociception by interacting with TRPA1 in the spinal cord. The findings that certain plant-derived cannabinoids and other non-electrophilic compounds cause concentration-dependent activation of mammalian TRPA1 show that covalent modification is not the only way to activate this ion channel [8] . We, therefore. investigated whether spinal activation of TRPA1 by a non-electrophilic Δ 9 -tetrahydrocannabinol derivative devoid of cannabinoid CB1 and CB2 receptor agonistic properties could be used to evoke antinociception. Here we show that activation of TRPA1 in the spinal cord by electrophilic APAP metabolites and the non-electrophilic cannabinoid Δ 9 -tetrahydrocannabiorcol reduces nociceptive behaviour in mice. The results indicate a new role of TRPA1 in synaptic signalling and disclose spinal TRPA1 activation as a novel antinociceptive mechanism that contributes to the analgesic activity of acetaminophen. The antinociceptive effect of APAP requires TRPA1 Previous in vivo studies have demonstrated that TRPA1-deficient mice have a reduced sensitivity in nociceptive tests using mechanical (paw-pressure and von Frey filaments) or cold stimuli, making these less suitable test modalities for the study of drug-induced antinociceptive mechanisms involving TRPA1 (refs 3 , 32 ; Supplementary Fig. S1 ). We therefore examined the importance of TRPA1 for the antinociceptive activity of APAP by measuring the latency to withdrawal from a 53°C hot plate and the number of abdominal constrictions after an intraperitoneal injection of acetic acid. These tests were chosen as the baseline responses did not differ between Trpa1 +/+ and Trpa1 −/− mice ( Fig. 1a,b ). Subcutaneous (s.c.) injection of APAP (300 mg kg −1 ), 1 h before the hot plate test, significantly increased the withdrawal latency in Trpa1 +/+ mice, but not in Trpa1 −/− mice ( Fig. 1a ). Similarly, pre-treatment with APAP (300 mg kg −1 , s.c.), 1 h before acetic-acid provocation, significantly reduced the number of constrictions in Trpa1 +/+ mice, but had no effect in Trpa1 −/− mice ( Fig. 1b ). 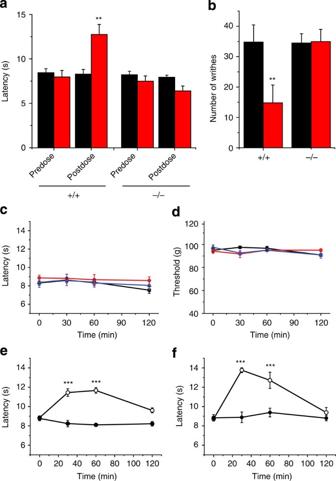Figure 1: TRPA1 is required for the antinociceptive effects of APAP. Subcutaneous injections of APAP 1 h before nociceptive tests (300 mg kg−1, red bars; vehicle in black bars) significantly increased the paw-withdrawal latency in the hot-plate test (a) and reduced the number of writhes in the acetic-acid writhing test (b) inTrpa1+/+mice, but not in theirTrpa1−/−littermates. Effect of intraplantar injections of APAP (vehicle in black, 100 μg in red and 500 μg in blue) on C57BL/6J mice behavioural responses in the hot-plate (c) and paw-pressure (d) tests. Effect of intrathecal injections of APAP (50 μg ineand 100 μg inf) in the hot-plate test inTrpa1+/+(empty circles) andTrpa1−/−mice (filled circles). Data show mean±s.e.m. for 6 mice per group. *P<0.05; **P<0.01 compared with vehicle group. ***P<0.001 compared with pre-injection latency. All data analysed by ANOVA followed by Tukey's HSD test. Figure 1: TRPA1 is required for the antinociceptive effects of APAP. Subcutaneous injections of APAP 1 h before nociceptive tests (300 mg kg −1 , red bars; vehicle in black bars) significantly increased the paw-withdrawal latency in the hot-plate test ( a ) and reduced the number of writhes in the acetic-acid writhing test ( b ) in Trpa1 +/+ mice, but not in their Trpa1 −/− littermates. Effect of intraplantar injections of APAP (vehicle in black, 100 μg in red and 500 μg in blue) on C57BL/6J mice behavioural responses in the hot-plate ( c ) and paw-pressure ( d ) tests. Effect of intrathecal injections of APAP (50 μg in e and 100 μg in f ) in the hot-plate test in Trpa1 +/+ (empty circles) and Trpa1 −/− mice (filled circles). Data show mean±s.e.m. for 6 mice per group. * P <0.05; ** P <0.01 compared with vehicle group. *** P <0.001 compared with pre-injection latency. All data analysed by ANOVA followed by Tukey's HSD test. Full size image APAP is thought to produce analgesia primarily by acting at central sites [10] , [11] , [12] and intraplantar injection of APAP (100 μg and 500 μg) had no effect on either hot plate latency or paw-pressure withdrawal threshold in wild-type mice ( Fig. 1c,d ). We therefore examined the effect of APAP administered intrathecally in the hot-plate test in Trpa1 +/+ and Trpa1 −/− mice. In good agreement with earlier studies that demonstrated a spinal site of action [15] , [16] , [17] , [18] , intrathecal APAP (50 and 100 μg) significantly increased the paw-withdrawal latency in wild-type mice on a 53°C hot plate ( Fig. 1e,f ). In contrast, APAP was without any antinociceptive activity in TRPA1-deficient littermates ( Fig. 1e,f ), indicating that TRPA1 is required for APAP activity in the hot-plate test when given intrathecally as well as following systemic administration. NAPQI and p -BQ activate TRPA1 Because our in vivo experiments demonstrated that TRPA1 is necessary for the antinociceptive activity of APAP, and that products of p -AP activate capsaicin-sensitive neurons ( Supplementary Fig. S2 ), we examined whether APAP or several of its metabolites ( Supplementary Fig. S3 ) can affect TRPA1 directly. APAP (1 μM–1 mM) and its deacetylation metabolite p -AP (100 nM–100 μM) failed to increase [Ca 2+ ] i in HEK293 cells expressing human TRPA1 ( Supplementary Fig. S4 ), demonstrating that these compounds are not TRPA1 agonists. Both compounds were also without antagonist activity against [Ca 2+ ] i responses evoked by the TRPA1 activator allyl isothiocyanate (AITC; Supplementary Fig. S4 ). TRPA1 is a sensory receptor for oxidants and thiol-reactive electrophilic compounds [6] , [7] , [8] , and APAP is metabolized in vivo to the highly reactive electrophilic compound NAPQI in humans and mice following therapeutic, non-toxic doses of APAP [19] , [24] , [26] . We, therefore, examined whether NAPQI can activate TRPA1 directly, using increases in [Ca 2+ ] i as a measure of TRPA1 activity. NAPQI evoked a concentration-dependent increase in [Ca 2+ ] i in CHO cells expressing either mouse TRPA1 or human TRPA1 with EC 50 values of 890±320 nM and 1,330±40 nM, respectively ( n =3–5, each experiment performed in triplicate; Fig. 2a ), in good agreement with a recent independent study [33] . We next used cultured dorsal root ganglion (DRG) neurons to study the agonist effects of NAPQI on sensory neurons and the importance of TRPA1 for any observed responses. NAPQI (500 nM) elicited [Ca 2+ ] i responses in 199 of 509 (39%) DRG neurons cultured from Trpa1 +/+ mice. In contrast, NAPQI only raised [Ca 2+ ] i in 2 of 521 neurons (0.4%) from Trpa1 −/− mice, demonstrating that NAPQI excites cultured sensory neurons through activation of TRPA1 ( Fig. 2b ). The effects of NAPQI were examined further using electrophysiological methods. In whole-cell voltage-clamp experiments, application of 500 nM NAPQI rapidly induced large currents in mouse TRPA1-expressing CHO cells with a current–voltage relationship typical of TRPA1 ( Fig. 2c ). These results demonstrate that NAPQI is a selective TRPA1 activator at concentrations in the submicromolar range. 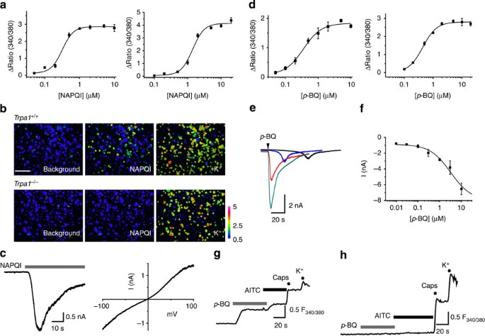Figure 2: NAPQI andp-BQ are potent TRPA1 activators. (a) Concentration-response relationship for [Ca2+]ielevations produced by NAPQI in cells expressing mouse TRPA1 (left panel) and human TRPA1 (right panel). Data points are mean±s.e.m. of triplicate wells. (b) Pseudocoloured images illustrating [Ca2+]iin DRG neurons before (background) and after challenges with NAPQI (500 nM) and 50 mM KCl. (c) Inward current activated by NAPQI (500 nM) in a mouse TRPA1–CHO cell (left panel) and the current–voltage relationship for TRPA1 stimulated by NAPQI (right panel). (d) Concentration-response curves for [Ca2+]iresponses produced byp-BQ in CHO cells expressing mouse TRPA1 (left panel) and human TRPA1 (right panel). Data points are mean±s.e.m. of triplicate wells. (e,f) Concentration-dependent amplitude and time course of currents elicited byp-BQ in mouse TRPA1-CHO cells (black trace 30 nM, blue 100 nM, red 300 nM and cyan 3 μM). Data infare mean±s.e.m. of three to six experiments for each concentration. (g,h) Typical examples of [Ca2+]iresponses in DRG neurons cultured fromTrpa1+/+(g) andTrpa1−/−mice (h) produced by challenges withp-BQ (1 μM), allyl isothiocyanate (50 μM), capsaicin (1 μM) and K+(50 mM). The scale bar represents 200 μm (b). Figure 2: NAPQI and p -BQ are potent TRPA1 activators. ( a ) Concentration-response relationship for [Ca 2+ ] i elevations produced by NAPQI in cells expressing mouse TRPA1 (left panel) and human TRPA1 (right panel). Data points are mean±s.e.m. of triplicate wells. ( b ) Pseudocoloured images illustrating [Ca 2+ ] i in DRG neurons before (background) and after challenges with NAPQI (500 nM) and 50 mM KCl. ( c ) Inward current activated by NAPQI (500 nM) in a mouse TRPA1–CHO cell (left panel) and the current–voltage relationship for TRPA1 stimulated by NAPQI (right panel). ( d ) Concentration-response curves for [Ca 2+ ] i responses produced by p -BQ in CHO cells expressing mouse TRPA1 (left panel) and human TRPA1 (right panel). Data points are mean±s.e.m. of triplicate wells. ( e , f ) Concentration-dependent amplitude and time course of currents elicited by p -BQ in mouse TRPA1-CHO cells (black trace 30 nM, blue 100 nM, red 300 nM and cyan 3 μM). Data in f are mean±s.e.m. of three to six experiments for each concentration. ( g , h ) Typical examples of [Ca 2+ ] i responses in DRG neurons cultured from Trpa1 +/+ ( g ) and Trpa1 −/− mice ( h ) produced by challenges with p -BQ (1 μM), allyl isothiocyanate (50 μM), capsaicin (1 μM) and K + (50 mM). The scale bar represents 200 μm ( b ). Full size image In addition to the oxidative formation of NAPQI, APAP is also converted to p -BQ in vivo ( Supplementary Fig. S3 ). p -BQ is another highly reactive electrophilic compound that is considerably more stable than NAPQI, making it more amenable to experimental investigation. p -BQ also acted as a TRPA1 agonist and evoked [Ca 2+ ] i responses in TRPA1-expressing CHO cells with EC 50 values of 360±20 nM and 440±20 nM for mouse TRPA1 and human TRPA1, respectively ( n =3–5, each experiment performed in triplicate; Fig. 2d ). In voltage-clamp experiments, p -BQ evoked TRPA1 current responses with concentration-dependent current amplitudes (EC 50 =3.2±0.6 μM) and rates of onset ( Fig. 2e,f ). To determine whether TRPA1 is required for sensory neuron responses to p -BQ, we used cultured DRG neurons from Trpa1 +/+ and Trpa1 −/− mice ( Fig. 2g,h ). In DRG neurons cultured from Trpa1 +/+ mice, 1 μM p -BQ produced [Ca 2+ ] i responses in 171 of 571 neurons (30%). The responding population of neurons was also sensitive to stimulation with AITC ( Fig. 2g ). In DRG cultures from Trpa1 −/− mice ( Fig. 2h ), p -BQ only increased [Ca 2+ ] i in 15 of 302 neurons (5%), and the few remaining p -BQ-sensitive neurons responded with a smaller increase in [Ca 2+ ] i than was seen in responsive neurons from Trpa1 +/+ mice. Expression of TRPA1 in the superficial dorsal horn Analysis of TRPA1 immunoreactivity in spinal cord sections from rat showed that TRPA1 is expressed in the superficial layers of the dorsal horn at various levels of the spinal cord ( Fig. 3a–e ). Co-localization studies showed that the TRPA1 immunoreactivity largely overlaps with that of TRPV1, calcitonin gene-related peptide and substance P, which are typical markers of nociceptive primary afferent neurons ( Fig. 3f ). Quantitative real-time PCR analysis did not detect any messenger RNA encoding TRPA1 and TRPV1 in the rat spinal cord ( C T values were 40±0.0 and 39±0.3 for TRPA1 and TRPV1, respectively; n =4), although analysis with TRPA1 and TRPV1 plasmids confirmed the ability of the assays to detect these transcripts ( C T values were 27±2.7 and 25±2.4 for TRPA1 and TRPV1, respectively; n =4). The same PCR assay detected both TRPA1 and TRPV1 transcripts in the rat bladder [34] . 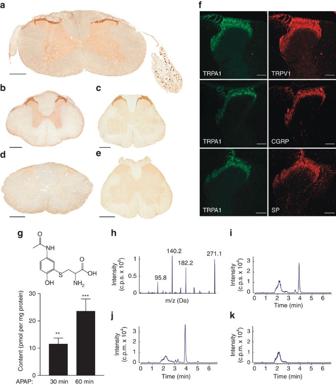Figure 3: TRPA1 and the acetaminophen metabolite NAPQI are present in the spinal cord. Immunohistochemical DAB staining displays TRPA1 immunoreactivity in the superficial layers of the dorsal horn at cervical (a), thoracic (b) and lumbar (c) levels of the rat spinal cord. No TRPA1 immunoreactivity is observed in the absence of primary antibody (d) or after co-incubation with primary antibody and blocking peptide (e). (f) The distribution of TRPA1 overlaps with that of TRPV1, calcitonin gene-related peptide (CGRP) and substance P (SP). The stable NAPQI metaboliteL-cysteinyl-S-acetaminophen is detected in the mouse spinal cord 30 min and 60 min after subcutaneous injection of 300 mg kg−1of acetaminophen (APAP;g). Mass spectrum ofL-cysteinyl-S-APAP obtained at positive mode [M+H]+=271.1 m/z; the fragmented ion m/z140.2 was selected for quantification ofL-cysteinyl-S-APAP (h). Chromatograms (m/z271.1>140.2) of mouse spinal cord samples spiked with 370 nM of the reference compoundL-cysteinyl-S-APAP (i) and 30 min afterin vivoadministration of APAP (j) or its vehicle saline (k). TheL-cysteinyl-S-APAP content was below the detection limit in vehicle-treated animals (k). Data show mean±s.e.m. for 6 mice per group. **P<0.01; ***P<0.001 compared with vehicle-treated animals (Mann–Whitney test). Scale bars represent 500 μm ina–e and 100 μm inf. Figure 3: TRPA1 and the acetaminophen metabolite NAPQI are present in the spinal cord. Immunohistochemical DAB staining displays TRPA1 immunoreactivity in the superficial layers of the dorsal horn at cervical ( a ), thoracic ( b ) and lumbar ( c ) levels of the rat spinal cord. No TRPA1 immunoreactivity is observed in the absence of primary antibody ( d ) or after co-incubation with primary antibody and blocking peptide ( e ). ( f ) The distribution of TRPA1 overlaps with that of TRPV1, calcitonin gene-related peptide (CGRP) and substance P (SP). The stable NAPQI metabolite L -cysteinyl- S -acetaminophen is detected in the mouse spinal cord 30 min and 60 min after subcutaneous injection of 300 mg kg −1 of acetaminophen (APAP; g ). Mass spectrum of L -cysteinyl- S -APAP obtained at positive mode [M+H] + =271.1 m/ z ; the fragmented ion m/ z 140.2 was selected for quantification of L -cysteinyl- S -APAP ( h ). Chromatograms (m/ z 271.1>140.2) of mouse spinal cord samples spiked with 370 nM of the reference compound L -cysteinyl- S -APAP ( i ) and 30 min after in vivo administration of APAP ( j ) or its vehicle saline ( k ). The L -cysteinyl- S -APAP content was below the detection limit in vehicle-treated animals ( k ). Data show mean±s.e.m. for 6 mice per group. ** P <0.01; *** P <0.001 compared with vehicle-treated animals (Mann–Whitney test). Scale bars represent 500 μm in a –e and 100 μm in f . Full size image L -cysteine conjugates of NAPQI and p -BQ in the spinal cord L -cysteinyl- S -APAP and L -cysteinyl- S- hydroquinone, the respective stable metabolites of NAPQI and p -BQ, were analysed in samples of mouse spinal cord as indicators of the formation of NAPQI and p -BQ. L -cysteinyl- S -APAP, but not L -cysteinyl- S- hydroquinone, was detected in the spinal cord 30 min and 60 min after subcutaneous injection of APAP at 300 mg kg −1 ( Fig. 3g,j ). As expected, L -cysteinyl- S -APAP was not detected in animals not given APAP ( n =6) or in time-matched, vehicle-treated animals ( Fig. 3k ). Intrathecal administration of NAPQI and p -BQ Next, we investigated the effect of intrathecal injections of the APAP metabolites NAPQI and p -BQ on behavioural nociceptive responses. We performed dose-response experiments with NAPQI and p -BQ administered in three different behavioural, nociceptive tests in mice—the hot-plate, paw-pressure and cold-plate tests. Both NAPQI and p -BQ produced a dose-dependent and reversible increase in the paw withdrawal latency in the hot-plate test in wild-type mice ( Fig. 4a,b ), but this effect was absent in Trpa1 −/− mice ( Fig. 4d,e ). Importantly, intrathecal injection of the well-known TRPA1 activator cinnamaldehyde (CA) produced a similar dose-dependent and reversible increase in the paw withdrawal latency in Trpa1 +/+ mice ( Fig. 4c ). A high dose (66 μg) of CA markedly increased the withdrawal latency in Trpa1 +/+ mice and, as seen with NAPQI and p -BQ, this antinociceptive effect was completely lost in Trpa1 −/− mice ( Fig. 4f ). 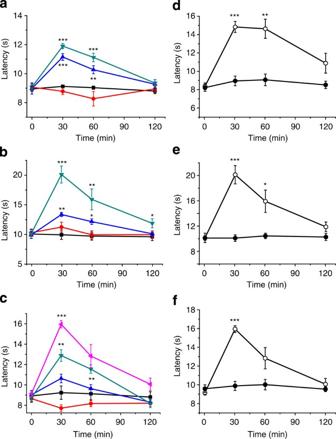Figure 4: Spinal antinociception evoked by NAPQI,p-BQ and CA. Dose-dependent effects of intrathecal injections of NAPQI (a; vehicle in black, 70 pg in red, 700 pg in blue and 7 ng in cyan),p-BQ (b; vehicle in black, 250 pg in red, 25 ng in blue and 2.5 μg in cyan) and cinnamaldehyde (c; vehicle in black, 6.6 ng in red, 66 ng in blue, 660 ng in cyan and 66 μg in magenta) on the paw-withdrawal threshold in the hot-plate test in lightly restrained C57BL/6J mice. Data show mean±s.e.m. for 6 mice per group. *P<0.05; **P<0.01; ***P<0.001 compared with time-matched vehicle group. Effect of intrathecal injections of NAPQI (d; 7 ng),p-BQ (e; 2.5 μg) and cinnamaldehyde (f; 66 μg) in the hot-plate test inTrpa1+/+mice (open circles) andTrpa1−/−mice (filled circles). Data show mean±s.e.m. for 6 mice per group. *P<0.05; **P<0.01; ***P<0.001 compared with pre-injection latency. All data analysed by ANOVA followed by Tukey's HSD test. Figure 4: Spinal antinociception evoked by NAPQI, p -BQ and CA. Dose-dependent effects of intrathecal injections of NAPQI ( a ; vehicle in black, 70 pg in red, 700 pg in blue and 7 ng in cyan), p -BQ ( b ; vehicle in black, 250 pg in red, 25 ng in blue and 2.5 μg in cyan) and cinnamaldehyde ( c ; vehicle in black, 6.6 ng in red, 66 ng in blue, 660 ng in cyan and 66 μg in magenta) on the paw-withdrawal threshold in the hot-plate test in lightly restrained C57BL/6J mice. Data show mean±s.e.m. for 6 mice per group. * P <0.05; ** P <0.01; *** P <0.001 compared with time-matched vehicle group. Effect of intrathecal injections of NAPQI ( d ; 7 ng), p -BQ ( e ; 2.5 μg) and cinnamaldehyde ( f ; 66 μg) in the hot-plate test in Trpa1 +/+ mice (open circles) and Trpa1 −/− mice (filled circles). Data show mean±s.e.m. for 6 mice per group. * P <0.05; ** P <0.01; *** P <0.001 compared with pre-injection latency. All data analysed by ANOVA followed by Tukey's HSD test. Full size image The effects of NAPQI and p -BQ were further examined in the paw-pressure and cold-plate tests where systemic administration of APAP exerts antinociceptive effects ( Fig. 5a,b ). Intrathecal injection of NAPQI and p -BQ produced dose-dependent increases in the withdrawal threshold in the paw-pressure test ( Fig. 5c,e ) and withdrawal latency in the cold-plate test in wild-type mice ( Fig. 5d,f ). As noted above, the greatly reduced paw-pressure and cold sensitivities of Trpa1 −/− mice normally precluded similar experiments in these mice. However, we were able to conduct one experiment in a group of Trpa1 −/− mice that showed slightly greater sensitivities than usual. Here a high dose of CA (66 μg) produced a marked antinociceptive effect in Trpa1 +/+ mice that was absent in Trpa1 −/− mice ( Supplementary Fig. S1 ). Taken together, the results show a spinal antinociceptive effect of electrophilic compounds in the paw-pressure and cold-plate tests that are likely to be mediated through activation of TRPA1. 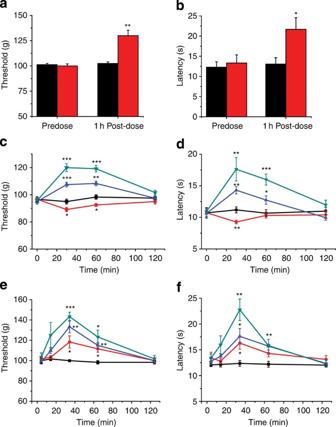Figure 5: APAP and its electrophilic metabolites are antinociceptive in the paw-pressure and cold-plate tests. APAP (300 mg kg−1, injected s.c. 1 h before tests) increased the paw-withdrawal threshold in the paw-pressure test (a) and paw-withdrawal latency in the cold-plate test (b) in C57BL/6J mice (vehicle in black, APAP in red). Dose-dependent effects of intrathecal injections of NAPQI (c,d; vehicle in black, 70 pg in red, 700 pg in blue and 7 ng in cyan) andp-BQ (e,f; vehicle in black, 250 pg in red, 25 ng in blue and 2.5 μg in cyan) in the paw-pressure test (c,e) and in the cold-plate test (d,f) in lightly restrained C57BL/6J mice. Data show mean±s.e.m. for 6 mice per group. *P<0.05; **P<0.01; ***P<0.001 compared with time-matched vehicle group (ANOVA followed by Tukey's HSD test). Figure 5: APAP and its electrophilic metabolites are antinociceptive in the paw-pressure and cold-plate tests. APAP (300 mg kg −1 , injected s.c. 1 h before tests) increased the paw-withdrawal threshold in the paw-pressure test ( a ) and paw-withdrawal latency in the cold-plate test ( b ) in C57BL/6J mice (vehicle in black, APAP in red). Dose-dependent effects of intrathecal injections of NAPQI ( c , d ; vehicle in black, 70 pg in red, 700 pg in blue and 7 ng in cyan) and p -BQ ( e , f ; vehicle in black, 250 pg in red, 25 ng in blue and 2.5 μg in cyan) in the paw-pressure test ( c , e ) and in the cold-plate test ( d , f ) in lightly restrained C57BL/6J mice. Data show mean±s.e.m. for 6 mice per group. * P <0.05; ** P <0.01; *** P <0.001 compared with time-matched vehicle group (ANOVA followed by Tukey's HSD test). Full size image NAPQI seemed to be more potent than p -BQ in the above in vivo experiments, which is in contrast to the apparent in vitro potencies of these agents. All experiments ( in vivo and in vitro ) with NAPQI and p -BQ were carried out as rapidly as possible to minimize the consequences of chemical instability. However, we cannot exclude that the purity differed between NAPQI batches (supplied by Toronto Research Chemicals or Sigma), although visual inspection did not reveal obvious differences between these batches. Furthermore, we noted that the in vitro activity of NAPQI in water solution declines with time, which is consistent with the observed effects being due to an action of the parent compound. We therefore consider it unlikely that decomposition products contribute to the effects seen with NAPQI. Δ 9 -Tetrahydrocannabiorcol activates TRPA1 On the basis of our previous findings that the cannabinoids Δ 9 -tetrahydrocannabinol ( 6 ) and cannabinol ( 13 ), which are non-electrophilic compounds, cause concentration-dependent activation of TRPA1 (ref. 4 ), we screened several plant-derived cannabinoids and synthetic Δ 9 -tetrahydrocannabinol derivatives for activity on mouse and human TRPA1 as well as for agonistic activity at human cannabinoid CB1 and CB2 receptors ( Supplementary Figs S5–S7 ). The compounds did not display any species differences with regard to TRPA1 activity ( Supplementary Figs S5 and S6 ). The structure-activity relationships for these compounds on human TRPA1 and human cannabinoid CB1 and CB2 receptors are summarized in Supplementary Figure S8 . Δ 9 -Tetrahydrocannabiorcol ( 16 ) displayed the highest activity on TRPA1 without affecting the cannabinoid receptors. When further characterized as a TRPA1 activator, Δ 9 -tetrahydrocannabiorcol was found to be as potent and effective as AITC in its ability to activate human TRPA1 expressed in HEK293 cells ( Fig. 6a ). The structure-activity is discussed in the Supplementary Discussion . 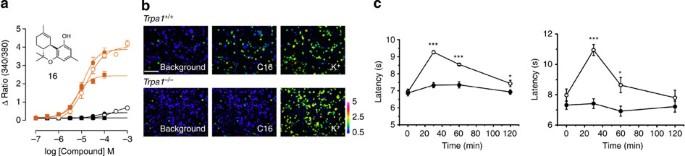Figure 6: Δ9-Tetrahydrocannabiorcol activates TRPA1 and causes spinal antinociception. (a) Application of Δ9-tetrahydrocannabiorcol (16, filled circles), allyl isothiocyanate (empty circles) and Δ9-tetrahydrocannabinol (filled squares) evoke concentration-dependent [Ca2+]iresponses in HEK293 cells expressing human TRPA1 (orange), but not in untransfected cells (black). Data show mean±s.e.m. of three to five experiments, each performed in triplicate. (b) In DRG neurons cultured fromTrpa1+/+mice, 20 μM Δ9-tetrahydrocannabiorcol produced [Ca2+]iresponses in 38% of the neurons. In DRG cultures fromTrpa1−/−mice, Δ9-tetrahydrocannabiorcol only increased [Ca2+]iin 3% of the neurons. (c) Intrathecal injections of Δ9-tetrahydrocannabiorcol (12 ng in left panel and 120 ng in right panel) significantly and reversibly increased the paw-withdrawal latency in the hot-plate test (53 °C) inTrpa1+/+mice (empty circles), but were without effect inTrpa1−/−animals (filled circles). Data show mean±s.e.m. for 6 mice per group. *P<0.05; ***P<0.001 compared with pre-injection latency (ANOVA followed by Tukey's HSD test). The scale bar represents 200 μm. Figure 6: Δ 9 -Tetrahydrocannabiorcol activates TRPA1 and causes spinal antinociception. ( a ) Application of Δ 9 -tetrahydrocannabiorcol ( 16 , filled circles), allyl isothiocyanate (empty circles) and Δ 9 -tetrahydrocannabinol (filled squares) evoke concentration-dependent [Ca 2+ ] i responses in HEK293 cells expressing human TRPA1 (orange), but not in untransfected cells (black). Data show mean±s.e.m. of three to five experiments, each performed in triplicate. ( b ) In DRG neurons cultured from Trpa1 +/+ mice, 20 μM Δ 9 -tetrahydrocannabiorcol produced [Ca 2+ ] i responses in 38% of the neurons. In DRG cultures from Trpa1 −/− mice, Δ 9 -tetrahydrocannabiorcol only increased [Ca 2+ ] i in 3% of the neurons. ( c ) Intrathecal injections of Δ 9 -tetrahydrocannabiorcol (12 ng in left panel and 120 ng in right panel) significantly and reversibly increased the paw-withdrawal latency in the hot-plate test (53 °C) in Trpa1 +/+ mice (empty circles), but were without effect in Trpa1 −/− animals (filled circles). Data show mean±s.e.m. for 6 mice per group. * P <0.05; *** P <0.001 compared with pre-injection latency (ANOVA followed by Tukey's HSD test). The scale bar represents 200 μm. Full size image The actions and selectivity of Δ 9 -tetrahydrocannabiorcol were further investigated on sensory neurons expressing native TRPA1. Δ 9 -Tetrahydrocannabiorcol (20 μM) elicited [Ca 2+ ] i responses in 123 of 328 (38%) DRG neurons cultured from Trpa1 +/+ mice, whereas it only raised [Ca 2+ ] i in 14 of 497 (3%) neurons obtained from Trpa1 −/− mice ( Fig. 6b ). The few remaining Δ 9 -tetrahydrocannabiorcol-sensitive neurons from Trpa1 −/− mice responded with a smaller increase in [Ca 2+ ] i than that seen in responsive neurons from Trpa1 +/+ mice. The stimulatory effects of Δ 9 -tetrahydrocannabiorcol are therefore primarily mediated by TRPA1. We next investigated whether non-covalent TRPA1 activation by Δ 9 -tetrahydrocannabiorcol would also result in antinociception. As shown in the hot-plate test, the antinociceptive effect of intrathecal administration of Δ 9 -tetrahydrocannabiorcol was evident in Trpa1 +/+ , but absent in Trpa1 −/− mice ( Fig. 6c ). Activation of TRPA1 inhibits ion currents in DRG neurons We next considered the possibility that activation of TRPA1 expressed on the central terminals of nociceptive DRG neurons inhibits the activity of voltage-gated calcium or sodium channels, thereby modifying synaptic transmission. Such mechanisms have previously been shown to operate following TRPV1 activation [35] , [36] , [37] , [38] , [39] . To assess the involvement of voltage-gated channels, we initially examined the effect of activation of TRPA1 on action potential properties and the excitability of DRG neurons in the current-clamp configuration. Action potentials evoked by current injections were recorded before and after a 1-min application of a relatively low concentration (500 nM) of p -BQ. In DRG neurons that did not depolarize when challenged with p -BQ (0.8±1.2 mV from a resting potential of −61±3, n =8), the action potential waveform was unchanged, and the rate of rise (10–90%) after p -BQ application was 103±6% ( n =8) of the original value ( Fig. 7a ). These findings demonstrated that p -BQ had no direct effect on neuronal excitability. In responsive neurons, application of p -BQ produced robust and slowly reversible depolarization (amplitude 42±5 mV from a resting potential of −63±3 mV, n =5; Fig. 7b ). As expected, it was not possible to evoke action potentials by current injection (up to 1 nA) in such depolarized neurons ( Fig. 7b ). After removal of p -BQ, the membrane potential returned to the original value (−64±4 mV), but the rate of rise (10–90%) of the action potential was significantly reduced to 47±4% ( n =5; P <0.001, Student's t -test) of the value observed before p -BQ application ( Fig. 7b ). Activation of TRPA1 also produced a shift in the threshold for action potential generation to more depolarized potentials (by 6±1.6 mV compared with 0±0.5 mV in p -BQ-insensitive neurons; P <0.001, Students t -test) and reduced the action potential overshoot by −12.9±5 mV (compared with 4.5±2 mV in p -BQ-insensitive neurons; P <0.01, Student's t -test). Some p -BQ-sensitive neurons had a pronounced hump on the falling phase of the action potential before stimulation with p -BQ ( Fig. 7b ). Following activation of TRPA1, the hump was dramatically reduced ( Fig. 7b ). The observed changes in action potential properties suggest that TRPA1 stimulation modified the activity of voltage-gated channels and prompted us to explore the effects of TRPA1 activation on sodium and calcium currents (I Na and I Ca ) in DRG neurons, using voltage-clamp methods. 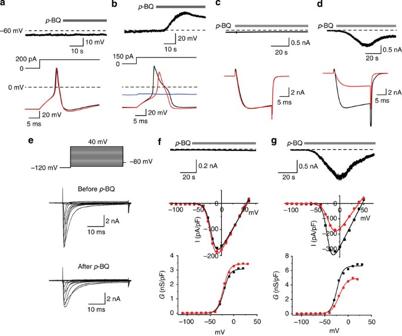Figure 7: TRPA1 activation reduces the excitability of DRG neurons. (a) Action potentials evoked by current injections before application (lower panel, black trace) and after washout ofp-BQ (red trace) in a neuron that did not depolarize in response to application of 500 nMp-BQ (upper trace). (b) Action potentials evoked by current injections (lower panel) in ap-BQ-responsive neuron (shown in upper trace) before application ofp-BQ (black trace), during thep-BQ evoked depolarization (blue trace) and after washout and complete repolarization (red trace). (c) Voltage-gated calcium currents (ICa) recorded in ap-BQ-insensitive (c) and ap-BQ-sensitive (d) DRG neuron before (lower panel, black trace) and after stimulation withp-BQ (red trace). ICawas evoked by a voltage step from −80 mV to 0 mV. (e) Voltage-gated sodium currents (INa) recorded before and after a challenge withp-BQ in ap-BQ-sensitive neuron. (f,g) Effect ofp-BQ on INadensity (middle panels) and conductance (bottom panels) in ap-BQ-insensitive (f) andp-BQ-sensitive neuron (g).p-BQ currents were recorded at a holding potential of −60 mV. Figure 7: TRPA1 activation reduces the excitability of DRG neurons. ( a ) Action potentials evoked by current injections before application (lower panel, black trace) and after washout of p -BQ (red trace) in a neuron that did not depolarize in response to application of 500 nM p -BQ (upper trace). ( b ) Action potentials evoked by current injections (lower panel) in a p -BQ-responsive neuron (shown in upper trace) before application of p -BQ (black trace), during the p -BQ evoked depolarization (blue trace) and after washout and complete repolarization (red trace). ( c ) Voltage-gated calcium currents (I Ca ) recorded in a p -BQ-insensitive ( c ) and a p -BQ-sensitive ( d ) DRG neuron before (lower panel, black trace) and after stimulation with p -BQ (red trace). I Ca was evoked by a voltage step from −80 mV to 0 mV. ( e ) Voltage-gated sodium currents (I Na ) recorded before and after a challenge with p -BQ in a p -BQ-sensitive neuron. ( f , g ) Effect of p -BQ on I Na density (middle panels) and conductance (bottom panels) in a p -BQ-insensitive ( f ) and p -BQ-sensitive neuron ( g ). p -BQ currents were recorded at a holding potential of −60 mV. Full size image In p -BQ-insensitive neurons, the amplitude of I Ca was unchanged after a challenge with p -BQ (I Ca after p -BQ was 96±4% of the initial amplitude, n =15; Fig. 7c ). However, in neurons that responded to p -BQ with an inward current typical of TRPA1 activation, the I Ca amplitude was sharply reduced to 31±9% of the initial amplitude ( n =8; P <0.001, Student's t -test; Fig. 7d ). Consistent with the lack of effect on action potentials in p -BQ-insensitive neurons, p -BQ did not alter I Na in such neurons ( Fig. 7f ) and had no effect on either the reversal (null current) potential (shift 0.5±0.8 mV, n =8), or on the maximal conductance (104±2% of pre- p -BQ value, n =8). In contrast, I Na was markedly reduced in p -BQ-responsive neurons ( Fig. 7e,g ). This p -BQ-induced reduction in I Na amplitude was explained in part by a significant shift in the reversal potential for Na + in the hyperpolarizing direction (shift −13±2.8 mV, n =5; P <0.001, Student's t -test; Fig. 7g ) and, in part, by a reduced maximal conductance (67±6% of pre- p -BQ value, n =5; P <0.001, Student's t -test; Fig. 7g ). In good agreement with the reduced excitability following TRPA1 activation noted in current-clamp recordings, the voltage required to elicit a half-maximal sodium conductance was shifted in the depolarizing direction after stimulation of TRPA1 (shift in V 1/2 =5.8±2.5 mV, n =5, compared with −0.8±0.7 mV in p -BQ-insensitive cells, n =8; Fig. 7f,g ). The observed shift in I Na reversal potential accurately reflects the reduced action potential overshoot and is consistent with an increase in [Na + ] i of 3–4 mM in response to p -BQ application. In the present study, we show for the first time that TRPA1 is required for the antinociceptive effects of intrathecally as well as systemically administered APAP, the most widely used over-the-counter analgesic and antipyretic agent. Notably, we found no effect of APAP when administered at the site of noxious stimulation in the periphery. Thus, our findings indicate that spinal TRPA1 has a crucial role in the antinociceptive action of APAP. Calcium imaging and electrophysiological experiments showed that although the electrophilic APAP metabolites NAPQI and p -BQ cause robust activation of heterologously expressed human and mouse TRPA1 and native ion channels in mouse DRG neurons, APAP and its non-electrophilic metabolite p -AP neither activate nor inhibit TRPA1. In vivo , intrathecal administration of either NAPQI or p -BQ elicited dose-dependent antinociception in the mouse paw-pressure and hot- and cold-plate assays, all of which are sensitive to systemic administration of the parent molecule APAP. Furthermore, the well-known TRPA1 activator CA was also able to produce antinociception when administered intrathecally in the mouse hot-plate test. As the effects of NAPQI, p -BQ and CA in this nociceptive test were absent in TRPA1-deficient mice, we demonstrate for the first time that activation of spinal TRPA1 can produce antinociception. TRPA1 is expressed in the soma and peripheral nerve endings of a subpopulation of TRPV1-containing peptidergic primary sensory neurons [1] , [34] , [40] . However, there is little information on the distribution of TRPA1 in the spinal cord. Our immunohistochemical analysis shows that TRPA1 is present in the dorsal horn at various levels of the rat spinal cord and that the distribution of TRPA1 is consistent with the termination of peptidergic primary afferents. We did not detect any TRPA1 transcripts in the rat spinal cord, which is also the case in the mouse spinal cord [1] . A recent study [9] reported that TRPA1 immunoreactivity disappeared in the rat lumbar spinal cord after dorsal rhizotomy, although immunoreactive postsynaptic dendrites were occasionally observed in the dorsal horn at an electron microscopic level. These findings suggest that TRPA1 expression in the spinal cord is largely restricted to the central projections of primary afferent neurons. In this context, it is interesting that several enzymes capable of oxidizing APAP, including CYP450 monoxygenase and COX, are present in the superficial laminae of the dorsal horn, suggesting that the TRPA1 active metabolites of APAP can be produced in the region of the central terminals of TRPA1-expressing sensory neurons [27] , [28] , [29] . Our detection of the stable NAPQI metabolite L -cysteinyl- S -APAP in the spinal cord after systemic administration of APAP is consistent with such a local metabolism of APAP to form reactive intermediates. A local metabolism of APAP could also explain why intrathecal administration of APAP produces antinociception, as demonstrated here and in other experimental studies [15] , [16] , [17] , [18] . The failure to find the p -BQ conjugate L -cysteinyl- S- hydroquinone in the spinal cord after systemic APAP treatment suggests that NAPQI is the major metabolite formed at this site. Intrathecal injection of electrophilic TRPA1 activators has recently been reported to elicit thermal hyperalgesia and mechanical allodynia in mice and neuropathic rats [41] , [42] , [43] . Interestingly, pharmacological inhibition of spinal TRPA1 attenuated mechanical hypersensitivity in various rodent models of subacute and chronic pain [43] , [44] , [45] . This is consistent with the observation that mechanical thresholds are elevated in Trpa1 −/− mice [3] , [32] . Our study shows that the outcome of spinal TRPA1 activation in intact animals is likely to depend on the degree of TRPA1 activation. We found that intrathecal administration of low doses of NAPQI and the TRPA1 activator CA could induce some degree of thermal hypersensitivity, whereas a pronounced antinociceptive effect was apparent at higher doses of these activators. Furthermore, we did not observe an initial nocifensive response with intrathecal doses of NAPQI, p -BQ or CA that produced clearcut antinociception in the various tests. Taken together, our data are consistent with a dominant antinociceptive effect of the metabolites after either systemic or intrathecal administration of APAP. The present observation that TRPA1 is involved in the antinociceptive effect of APAP together with our finding that APAP can undergo FAAH-dependent conversion to N -acylphenolamines, which produce antinociception via activation of TRPV1 in the brain [22] , [23] , shows that the mechanism of action of APAP is complex. This is not surprising, considering the extensive metabolism of APAP in both animals and man. Thus, depending on the dose and route of administration, the nociceptive test and species used, TRPA1 and TRPV1 may each contribute to various extents to the antinociceptive effect of APAP. However, further studies are needed to clarify the relative contribution of these mechanisms. Nevertheless, by studying the pharmacology of APAP, we have disclosed a new antinociceptive mechanism, driven by activation of TRPA1 in the spinal cord, which could be explored for developing novel analgesics. Whether activation of TRPA1 contributes to the action of other existing analgesics, such as some of the nonsteroidal anti-inflammatory fenamates [46] , [47] , remains to be studied. Our findings that activation of TRPA1 produced an initial 'depolarization block' and an extensive and sustained inhibition of voltage-gated calcium and sodium currents in DRG neurons provide a mechanism for the antinociceptive effect of spinal TRPA1 activation. This is in line with previous studies, showing that activation of TRPV1 produces a sustained inhibition of voltage-gated calcium and sodium channels [35] , [36] , [37] , [38] , [39] in sensory neurons as well as spinal antinociception [30] , [31] , [48] . On the basis of these studies, a model for TRPA1-mediated inhibition of synaptic transmission emerges, in which sodium and calcium influx through TRPA1 produces an initial depolarization-induced inactivation of voltage-gated sodium channels and a sustained inhibition of voltage-gated sodium and calcium currents, reducing action potential-dependent neurotransmitter release ( Fig. 8 ). Such a mechanism can also explain the observations that activation of TRPA1 in rat spinal cord slices inhibits C-fibre-evoked excitatory postsynaptic currents, while increasing spontaneous excitatory postsynaptic currents in substantia gelatinosa neurons [49] , [50] , [51] . 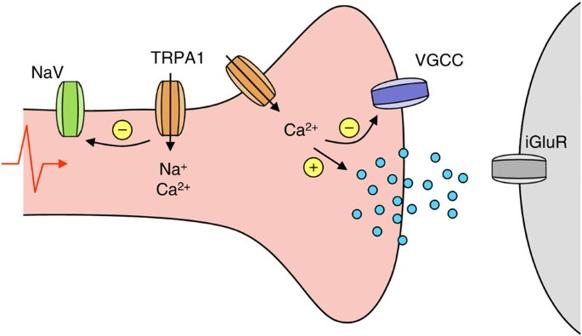Figure 8: Consequences of spinal TRPA1 activation. TRPA1 is expressed on the central terminals of primary sensory neurons in the dorsal horn of the spinal cord. Activation of TRPA1, for example, by electrophilic metabolites of APAP, increases the influx of calcium, which causes inactivation of voltage-gated calcium channels (VGCC)35,36. Cation influx through TRPA1 also depolarizes the membrane and produces a sustained inhibition of voltage-gated sodium channels (NaV), thereby reducing neuronal excitability and action potential-dependent neurotransmitter release. The net result of these actions is inhibition of C-fibre-evoked postsynaptic excitation, although TRPA1-mediated calcium influx may initially increase spontaneous excitatory postsynaptic currents via activation of ionotropic glutamate receptors (iGluR)42,49,50,51. Similar molecular mechanisms have been advanced to explain the antinociceptive effect of spinal TRPV1 activation31,48. Figure 8: Consequences of spinal TRPA1 activation. TRPA1 is expressed on the central terminals of primary sensory neurons in the dorsal horn of the spinal cord. Activation of TRPA1, for example, by electrophilic metabolites of APAP, increases the influx of calcium, which causes inactivation of voltage-gated calcium channels (VGCC) [35] , [36] . Cation influx through TRPA1 also depolarizes the membrane and produces a sustained inhibition of voltage-gated sodium channels (NaV), thereby reducing neuronal excitability and action potential-dependent neurotransmitter release. The net result of these actions is inhibition of C-fibre-evoked postsynaptic excitation, although TRPA1-mediated calcium influx may initially increase spontaneous excitatory postsynaptic currents via activation of ionotropic glutamate receptors (iGluR) [42] , [49] , [50] , [51] . Similar molecular mechanisms have been advanced to explain the antinociceptive effect of spinal TRPV1 activation [31] , [48] . Full size image It is noteworthy that APAP has not been replaced therapeutically by any analogue that is not metabolized to reactive molecules. This would support the idea that the effect of APAP is mediated by its electrophilic metabolites. Ingestion of higher doses of APAP to increase the local formation of electrophiles, or administration of an electrophilic TRPA1 activator to produce antinociception are potentially tissue damaging. It is therefore of interest that TRPA1 can be activated by non-electrophilic compounds, such as Δ 9 -tetrahydrocannabinol, menthol, clotrimazole and dihydropyridines [8] . However, these particular compounds cannot be used to address whether non-electrophilic activation of TRPA1 also produces spinal antinociception, because they also interact with other targets in the nociceptive pathway. Therefore, on the basis of the structure of Δ 9 -tetrahydrocannabinol, we synthesized and selected plant-derived cannabinoids that activated TRPA1, but were inactive at cannabinoid CB1 and CB2 receptors to exclude antinociceptive effects evoked by stimulation of cannabinoid receptors. Using this screening strategy, we identified Δ 9 -tetrahydrocannabiorcol as an appropriate tool to investigate whether covalent activation of TRPA1 is critical for its antinociceptive action in the spinal cord. Our in vivo studies clearly demonstrated that this is not the case, as intrathecal administration of Δ 9 -tetrahydrocannabiorcol produced TRPA1-mediated antinociception in the mouse hot-plate test. In summary, this study shows that the APAP metabolites NAPQI and p -BQ, which are powerful TRPA1 activators, produce a TRPA1-mediated spinal antinociception in mice. We provide evidence that NAPQI is present in the spinal cord after systemic administration of APAP and suggest that this electrophilic metabolite through activation of TRPA1 on central terminals of primary afferents contributes to the antinociceptive effect of APAP. The ability of Δ 9 -tetrahydrocannabiorcol, a non-electrophilic Δ 9 -tetrahydrocannabinol derivative, to produce TRPA1-mediated spinal antinociception demonstrates that pharmacological activation of this ion channel by non-tissue damaging compounds could be a novel pharmacological strategy for treatment of pain. Behavioural studies Animal studies were performed according to the UK Home Office Animal Procedures Act (1986) after in-house ethical review. Data shown are from female C57BL/6J mice or from male and female homozygote Trpa1 −/− and Trpa1 +/+ littermates. C57BL/6J mice were obtained from Harlan UK. TRPA1-null mice and wild-type littermates were bred from heterozygotic mice provided by Drs Kelvin Kwan and David Corey (Harvard Medical School, Boston, MA) [3] . Vehicle (saline) or APAP (300 mg kg −1 ) were administered by subcutaneous injection (5 ml kg −1 bodyweight) into the scruff of the neck 1 h before induction of nociceptive responses triggered by acetic acid, or thermal or mechanical stimuli. Intrathecal injections were carried out in fully conscious manually restrained mice. A 30-gauge needle attached to a 25 μl Hamilton syringe was inserted through the skin, between the L5–L6 vertebrae and into the subarachnoid space and a volume of 5 μl was slowly injected. NAPQI was dissolved initially in dimethylsulphoxide and then rapidly diluted to 10% dimethylsulphoxide in 0.9% saline for injection within 3–4 min of dissolution. APAP and p -BQ was prepared directly in saline and CA was dissolved in 0.5% Tween 80 in saline. The nociceptive tests are described in detail in the Supplementary Methods . Cell culture CHO and HEK293 cells as well as DRG neurons were cultured as described in the Supplementary Methods . Imaging of intracellular calcium levels DRG neurons were loaded with 2 μM Fura-2 AM (Molecular Probes) in the presence of 1 mM probenecid for ~1 h. The dye loading and the subsequent experiments were performed in a physiological saline solution, containing (in mM) 140 NaCl, 5 KCl, 10 glucose, 2 CaCl 2 , 1 MgCl 2 and 10 HEPES, buffered to pH 7.4 (with NaOH). Compounds were applied to neurons by continuous local microperfusion of solution through a fine tube placed close to the cells being studied. Experiments were conducted at 30 °C. Images of a group of cells were captured every 2 sec (340 and 380 nm excitation wavelengths, 520 nm emission wavelength), using a microscope-based imaging system (PTI). Analyses of emission intensity ratios at 340 nm/380 nm excitation ( R , in individual cells) were performed, using the ImageMaster suite of software. In some experiments, changes in intracellular calcium ([Ca 2+ ] i ) were determined in CHO or HEK293 cells grown in 96-well black walled plates (Costar), using a Flexstation 3 (Molecular Devices). Cells were loaded with Fura 2-AM and assays were carried out at 25 °C. Basal emission ratios with excitation wavelengths of 340 nm and 380 nm were measured and changes in dye emission ratio determined at various times after compound addition. Electrophysiology CHO cells expressing mouse TRPA1 and rat DRG neurons were studied under voltage-clamp and current-clamp conditions, using an Axopatch 200B amplifier and pClamp 10 software (Axon Instruments). Whole-cell currents were recorded at a holding potential of −60 mV unless stated otherwise. Drugs and solutions were applied by local superfusion, using a rapid solution changer (Bio-Logic). Borosilicate glass pipettes (2–5 MΩ, 75–80% series resistance compensation) were filled with (in mM) 140 KCl, 1 CaCl 2 , 2 MgATP, 10 EGTA and 10 HEPES, buffered to pH 7.4 (with KOH), for studies on agonist-evoked currents where the external solution was as described above for [Ca 2+ ] i measurements. Voltage-activated calcium currents were studied in an extracellular solution that contained (in mM) 140 Choline Cl, 1 MgCl 2 , 5 CaCl 2 , 10 glucose and 10 HEPES, titrated to pH 7.4 (with CsOH). The recording electrodes for these experiments were filled with 140 CsCl, 2 MgATP, 1 CaCl 2 , 10 EGTA and 10 HEPES, titrated to pH 7.4 (with CsOH). Sodium currents were recorded using an external solution, containing 100 Choline Cl, 50 NaCl, 20 TEACl, 5MgCl 2 , 0.01 CaCl 2 and 10 HEPES, titrated to pH 7.4 (with NaOH). The internal solution contained (in mM) 135 CsCl, 5 NaCl, 2 MgATP, 1 CaCl 2 and 10 EGTA, titrated to pH 7.4 (with CsOH). In the studies of voltage-gated sodium and calcium currents, p -BQ was applied in the solution described for [Ca 2+ ] i measurements. Current-clamp recordings were performed in the external solution used for [Ca 2+ ] i measurements and the internal solution contained (in mM) 135 KCl, 5 NaCl, 2 MgATP, 1 CaCl 2 , 10 EGTA and 10 HEPES, titrated to pH 7.4 (with KOH). Excitability measurements were performed by injecting DRG neurons with depolarizing current pulses in increments of 50 pA (50 ms duration) from 50 to 1,000 pA. The minimal current injection sufficient to evoke an action potential in each neuron was used for analysis of action potential properties. Immunohistochemistry Male and female Sprague–Dawley rats (225 g; Taconic) were anaesthetized with pentobarbitone and transcardially perfused with saline for 5–10 min, followed by 4% paraformaldehyde in 0.1 M phosphate buffer for 10 min. Spinal cords were removed and post-fixed in the same fixative overnight at 4 °C, and subsequently cryopreserved in 15% sucrose for 2 days. Tissues were frozen with isopentane and cut into 25 μm thick sections, preincubated with a phosphate buffer solution, containing 0.2% Triton X-100 and 0.1% bovine serum albumin, for 2 h before incubation overnight with the primary antibodies as further described in Supplementary Methods . The Aperio Scanscope system was used to scan and visualize DAB-stained tissues (LRI Instrument AB). Fluorescence microscopy was performed with an Eclipse TE2000-S confocal microscope (Nikon) and images were acquired with the software program EZ–C1 gold version 3.0 version. Quantitative real-time PCR Total RNA was isolated with Trizol from the spinal cord of four rats and used to synthesize complementary DNA for quantitative real-time PCR analyses. All samples were analysed as triplicates. The housekeeping-gene β-actin (rat) was used as an internal reference. The cycle threshold ( C T ) value for the house-keeping gene β-actin (internal reference) was 32±1.8. C T values below 40 were considered positive. The following TaqMan gene expression assays from Applied Biosystems were used (assay ID): TRPV1 (Rn 00583117_m1), TRPA1 (Rn01473803_m1) and β-actin (4352931E). Quantification of Metabolites These studies were approved by the Malmö/Lund animal ethics committee. Male and female C57BL/6 mice (20–30 g; Taconic) were treated with acetaminophen (300 mg kg −1 ) or vehicle (saline), each given subcutaneously into the scruff of the neck at a volume of 10 ml kg −1 bodyweight. The animals were sacrificed 30 min or 60 min post dose by cervical dislocation under light isofluran anaesthesia. The spinal column was transected at the upper cervical and lumbar levels. A cannula was inserted into the caudal end of the spinal canal. The spinal cord was then pneumoejected through the cervical orifice and snap frozen in liquid nitrogen. The ejected spinal cord, weighing ~40 mg, was homogenized in 200 μl of ice-cold Tris buffer (10 mM; pH 7.6), containing 1 mM of EDTA. Aliquots (200 μl) of homogenates were precipitated with 1 ml ice-cold acetone, containing d 3 - L -cysteinyl- S -APAP (2 μM) and d 3 - L -cysteinyl- S -hydroquinone (2 μM) as internal standards. After centrifugation at 25,200 g for 20 min (4 °C), the supernatants were collected in polypropylene tubes and vacuum evaporated. The extraction residues were reconstituted in 200 μl of a mixture of formic acid (0.45%) and methanol (10%). The pellet was saved for determination of protein content. Samples were analysed as further described in Supplementary Methods . The within-day reproducibility, determined at a concentration of 10 μM, was 2.8 and 3.3% ( n =69) for L -cysteinyl- S -APAP and L -cysteinyl- S -hydroquinone, respectively. The synthesis of the metabolites is described in the Supplementary Methods . Synthesis of cannabinoids Two general methods were used to synthesize the various cannabinoid derivatives. Cannabinoids substituted on phenolic ring: resorcinol derivatives were added to a solution of (+)- p -menth-2-ene-1,8-diol acetate in dry dichloromethane. Cannabinoids substituted on cyclohexene ring: unsaturated aldehyde derivatives were added to olivetol in dry toluene in the presence of Et 2 AlCl. For full details, see Supplementary Methods . Cannabinoid receptor-mediated inhibition of cAMP accumulation To screen for CB1 and CB2 receptor agonistic properties of the cannabinoid derivatives, we used the established CB1/CB2-cAMP assay. The effect of cannabinoid derivatives and vehicle on forskolin-stimulated (10 μM) cAMP accumulation was determined after drug exposure for 20 min. The reaction was stopped by addition of one volume ice-cold 0.2 M HCl, and cAMP was determined by radioimmunoassay. The responses to test compounds are presented as a percentage of the forskolin-induced cAMP accumulation in the presence of vehicle ( 5% ethanol). For full details, see Supplementary Methods . How to cite this article: Andersson, D. A. et al . TRPA1 mediates spinal antinociception induced by acetaminophen and the cannabinoid Δ 9 -tetrahydrocannabiorcol. Nat. Commun. 2:551 doi: 10.1038/ncomms1559 (2011).